A germanate transparent conductive oxide Wide bandgap conductors such as In 2 O 3 and ZnO are used as transparent conducting oxides (TCOs). To date, TCOs are realized using post transition metal cations with largely spread s -orbitals such as In 3+ , Sn 4+ , Zn 2+ and Cd 2+ . On the other hand, no good electronic conductor has been realized in oxides of Al, Si and Ge. Here we report the conversion of an oxide of Ge into a good electronic conductor by employing the concept of superdegeneracy. We find that cubic SrGeO 3 , synthesized under high pressure, displays a direct bandgap of 3.5 eV, a carrier mobility of 12 cm 2 (Vs) −1 , and conductivities of 3 Scm −1 (DC) and 400 Scm −1 (optical conductivity). This is the first Ge-based electronic conductive oxide, and expands the family of TCOs from ionic oxides to covalent oxides. Transparent conducting oxides (TCOs) [1] , which have a high electrical conductivity and a high optical transparency in visible light, are necessary for a variety of optoelectronic applications. However, high conductivity materials are generally not optically transparent. To date, metal elements such as In, Sn, Zn and Cd ('TCO-cations') are essential for TCO formation and form a frontier in the periodic table that separates themselves from the insulating elements such as Al, Si and Ge (the only exception is 12CaO·7Al 2 O 3 with a special nanocage structure [2] ). These TCO-cations are post-transition metal cations with electronic configurations of ( n −1)d 10 n s 0 ( n is the principal quantum number and should be ≥4 to obtain good electrical conductivities) [3] , [4] , [5] . The spherical spread vacant s orbitals of these metal cations form highly dispersed conduction bands (CBs) with small effective electron masses, and consequently contributes to high electron mobilities. New TCO materials such as MgIn 2 O 4 have been developed based on this guideline [6] , [7] , [8] . However, it is difficult to create a TCO based on the metal cations that are located in the upper right part of the periodic table, because the spatial spread of their vacant s orbitals is small. The small CB dispersion results in a large effective mass and this raises the energy levels of the CB minimum (CBM), which makes electron doping difficult. In reality, sufficient electronic conduction has yet been obtained for the oxides of metals such as Al, Si and Ge. Herein, we show that cubic-SrGeO 3 with the perovskite-type structure ( Fig. 1a ) is the first Ge-based transparent electronic conductor. This achievement proposes a new design concept for covalent TCOs, which realizes a deep CBM because of superdegeneracy that appears in high-symmetry crystals of a highly covalent nature. 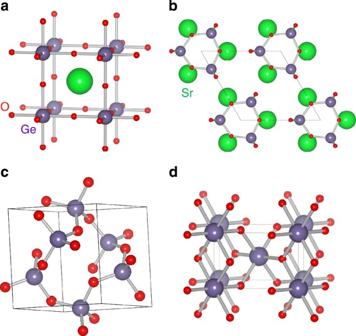Figure 1: Crystal structures of Ge oxides. (a) HP-SrGeO3with cubic perovskite type. (b) AP-SrGeO3composed of isolated rings23,24. (c) AP-GeO2has a complex α-quartz type structure25. (d) HP-GeO2takes rutile-type composed of GeO6octahedra26. Figure 1: Crystal structures of Ge oxides. ( a ) HP-SrGeO 3 with cubic perovskite type. ( b ) AP-SrGeO 3 composed of isolated rings [23] , [24] . ( c ) AP-GeO 2 has a complex α-quartz type structure [25] . ( d ) HP-GeO 2 takes rutile-type composed of GeO 6 octahedra [26] . Full size image Sample structures Powder samples of undoped and La-doped SrGeO 3 ((Sr 0.95 La 0.05 )GeO 3 ) were synthesized at ambient pressure (AP). 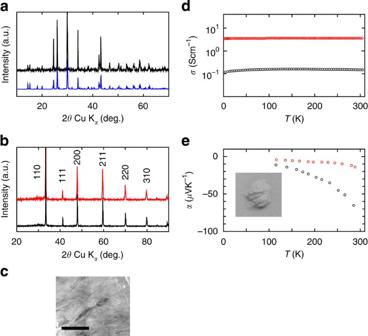Figure 2: Powder X-ray diffraction (XRD) patterns and electrical properties. (a) Measured powder XRD pattern of the SrGeO3sample synthesized at AP (black symbols) along with its simulation pattern (blue symbols). (b) Measured powder XRD patterns of the undoped (black symbols) and La-doped SrGeO3samples (red symbols) after the HP treatment. (c) SEM image of polished surface of HP-SrGeO3pellet. Scale bar shows 3 μm. (d) Temperature dependence of the electrical conductivities and (e) Seebeck coefficients for the undoped (black symbols) and the La-doped HP-SrGeO3(red symbols). Inset toeshows a photograph of the undoped HP-SrGeO3powder. These samples were identified as the AP-SrGeO 3 phase by powder X-ray diffraction, as shown in Figure 2a . It has a monoclinic lattice and is composed of an isolated (GeO 4 ) ring structure ( Fig. 1b ). A high-pressure (HP) treatment at 5.5 GPa and 1,100 °C converted these structures to cubic-SrGeO 3 (HP-SrGeO 3 ) with perovskite type [9] ( Fig. 1a ), as shown in Figure 2b (a photograph of the material is shown in the inset of Fig. 2e ). The observed dense microstructure of the polished surface of the pellet, shown in a scanning electron microscopic (SEM) image in Figure 2c enables us the optical reflectance measurements, as well as carrier transport experiments. Figure 2: Powder X-ray diffraction (XRD) patterns and electrical properties. ( a ) Measured powder XRD pattern of the SrGeO 3 sample synthesized at AP (black symbols) along with its simulation pattern (blue symbols). ( b ) Measured powder XRD patterns of the undoped (black symbols) and La-doped SrGeO 3 samples (red symbols) after the HP treatment. ( c ) SEM image of polished surface of HP-SrGeO 3 pellet. Scale bar shows 3 μm. ( d ) Temperature dependence of the electrical conductivities and ( e ) Seebeck coefficients for the undoped (black symbols) and the La-doped HP-SrGeO 3 (red symbols). Inset to e shows a photograph of the undoped HP-SrGeO 3 powder. Full size image Electrical properties Figure 2d,e show the temperature dependence of the electrical conductivities and the Seebeck coefficients for the undoped and the La-doped HP-SrGeO 3 samples. The electrical conductivities are nearly temperature independent. Also, the Seebeck coefficients are negative for both the samples, which indicates that these were degenerate n -type conductors. The DC conductivity, σ DC , at 300 K for the La-doped sample was 3 Scm −1 , being consistent with the smaller Seebeck coefficients and the smaller temperature dependence than those of the undoped HP-SrGeO 3 . 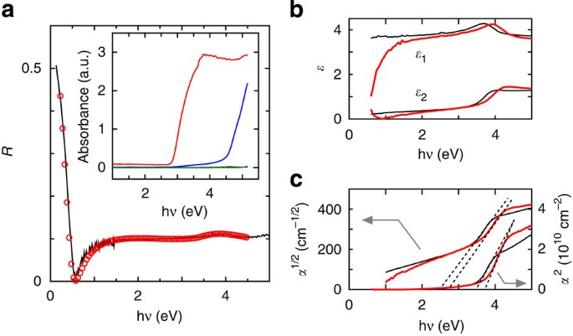Figure 3: Bandgaps of HP-SrGeO3and related germanium oxides. (a) Reflectance spectra of La-doped HP-SrGeO3. The solid line shows the measured data and the red circles show the simulated result using the Drude–Tauc–Lorentz combined model. The inset shows the diffuse reflectance spectra of the powder samples of undoped AP-GeO2(the green line), HP-GeO2(blue), AP-SrGeO3(completely overlapped with the data of AP-GeO2, the green line) and HP-SrGeO3(red). (b) Dielectric functions and (c) absorption spectra for undoped (the black lines) and La-doped HP-SrGeO3(the red lines) obtained by spectroscopic ellipsometry. The absorption spectra are plotted for the direct and indirect transition-type semiconductors. Optical properties and optical conductivity Figure 3 shows optical reflectance spectra, complex dielectric functions ( ɛ *( ω )= ɛ 1 ( ω )+ jɛ 2 ( ω ), where j denotes the imaginary unit), and absorption spectra of the Ge oxides discussed in this paper. From the absorbance spectra shown in the inset of Figure 3a , it is evident that HP-GeO 2 and HP-SrGeO 3 have smaller bandgaps than the AP phases. The sharp increase in reflectance at <0.5 eV can be reproduced using the Drude model with a plasma frequency of 1.0 eV and a momentum relaxation time of 2.0 fs, which substantiates that HP-SrGeO 3 has high-density free electrons in the CB. The optical conductivity ( σ opt ( ω )≡ ωɛ 2 ( ω )) at the DC limit, σ opt ( ω =0), of 410 Scm −1 was obtained from this fitting. The carrier density ( N opt ) and mobility ( μ opt ) can be determined from these results by assuming a reasonable electron effective mass, m e *. In many TCOs, the effective electron masses range between 0.25–0.35 m e (m e denotes the rest mass of the electron) [10] . Assuming m e *=0.3 m e , we obtained N opt =2.2×10 20 cm −3 and μ opt =11.6 cm 2 (Vs) −1 . We needed to incorporate a 75 nm thick surface insulating layer to reproduce the dip structure that occurs at 0.55 eV, which suggests that the mobile electrons are annihilated in the thin surface region. Figure 3: Bandgaps of HP-SrGeO 3 and related germanium oxides. ( a ) Reflectance spectra of La-doped HP-SrGeO 3 . The solid line shows the measured data and the red circles show the simulated result using the Drude–Tauc–Lorentz combined model. The inset shows the diffuse reflectance spectra of the powder samples of undoped AP-GeO 2 (the green line), HP-GeO 2 (blue), AP-SrGeO 3 (completely overlapped with the data of AP-GeO 2 , the green line) and HP-SrGeO 3 (red). ( b ) Dielectric functions and ( c ) absorption spectra for undoped (the black lines) and La-doped HP-SrGeO 3 (the red lines) obtained by spectroscopic ellipsometry. The absorption spectra are plotted for the direct and indirect transition-type semiconductors. Full size image Electronic structure The bandgap values were obtained from an analysis of the spectroscopic ellipsometry data shown in Figure 3b,c . The ɛ 2 ( ω ) values show clear absorption structures at >3 eV for the undoped and the La-doped SrGeO 3 . For undoped and La-doped SrGeO 3 , the indirect bandgaps ( E g,indir ), which were estimated from the α 0.5 –hν plots, were 2.70 and 2.80 eV, respectively. The direct bandgaps ( E g,dir ) estimated from the α 2 –hν plots were 3.45 and 3.70 eV, respectively. We used density functional theory to explain the high electrical conductivity of HP-SrGeO 3 . 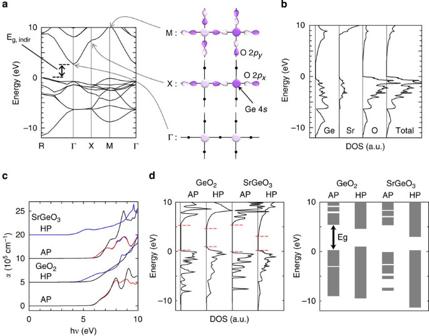Figure 4: Calculated electronic structures of germanium oxides. (a) Band structure and illustrations of the corresponding chemical bonds for HP-SrGeO3. The light and dark purple areas indicate positive and negative phases of the wave functions, respectively. The dots indicate atoms that do not contribute to the chemical bonds. (b) Total and projected DOSs (O, Sr and Ge) for HP-SrGeO3. Those of Sr and Ge are expanded by a factor of 5. (c) Calculated optical absorption spectra for AP-GeO2, HP-GeO2, AP-SrGeO3and HP-SrGeO3. αxx, αyyand αzzare represented by the blue, red and black lines, respectively. Each spectrum is shifted by 5×105cm−1for clarity. (d) Total DOSs and simplified band alignment for the four Ge-based oxides. The energy is aligned by the O 2 s levels (−17 to −21 eV below their respective EVBM's). The DOSs of the unoccupied states of HP-SrGeO3are magnified by a factor of 5. The band edges are shown by the red dashed lines. Figure 4a shows the band structure of HP-SrGeO 3 that indicates that HP-SrGeO 3 is a semiconductor with an indirect bandgap of 2.7 eV. Figure 4b shows the projected density of states (DOS) for HP-SrGeO 3 . Vacant Sr orbitals do not contribute to the bandgap because their contribution appears only at >8 eV, which is much higher than the CBM (located at +2.7 eV). It is thus obvious that HP-SrGeO 3 is a Ge-based electronic conductor. The calculated optical absorption spectra and the DOSs of Ge oxides are shown in Figure 4c,d , respectively. The calculated absorption edge energies agree well with the experimental absorbance spectra shown in the inset of Figure 3a . However, a large discrepancy between the calculated absorption edge (3.3 eV) and bandgap (2.7 eV, extracted from the band structure in Fig. 4a ) is found for HP-SrGeO 3 . Figure 4: Calculated electronic structures of germanium oxides. ( a ) Band structure and illustrations of the corresponding chemical bonds for HP-SrGeO 3 . The light and dark purple areas indicate positive and negative phases of the wave functions, respectively. The dots indicate atoms that do not contribute to the chemical bonds. ( b ) Total and projected DOSs (O, Sr and Ge) for HP-SrGeO 3 . Those of Sr and Ge are expanded by a factor of 5. ( c ) Calculated optical absorption spectra for AP-GeO 2 , HP-GeO 2 , AP-SrGeO 3 and HP-SrGeO 3 . α xx , α yy and α zz are represented by the blue, red and black lines, respectively. Each spectrum is shifted by 5×10 5 cm −1 for clarity. ( d ) Total DOSs and simplified band alignment for the four Ge-based oxides. The energy is aligned by the O 2 s levels (−17 to −21 eV below their respective E VBM 's). The DOSs of the unoccupied states of HP-SrGeO 3 are magnified by a factor of 5. The band edges are shown by the red dashed lines. Full size image HP-SrGeO 3 is the first Ge-based transparent electronic conductor with a bandgap of 3.5 eV, although Ge oxides are typical insulators with wide bandgaps (>5 eV). The HP-SrGeO 3 is a well-known phase for geophysicists and has been investigated extensively from geophysical interests [11] ; however, no cultivation of electronic functions has, to our knowledge, been examined so far. To understand the peculiar properties of HP-SrGeO 3 , we, first, survey the characteristic features of the electronic structures of the Ge oxides. Ge ions in most of the Ge oxides synthesized at AP take tetrahedral GeO 4 sites as shown in Figure 1b,c , and have large bandgaps (the inset to Fig. 3a ). The insulating nature of AP-GeO 2 with the α-quartz type structure ( Fig. 1c ) originates from the large bandgap (5.1 eV) [12] and its structural flexibility. In this structure, two (GeO 4 ) tetrahedra are connected through a twofold coordinated O ion. The tetrahedral GeO 4 is composed of highly covalent Ge–O bonds, and this twofold oxygen bridging structure, (GeO 4 )–(GeO 4 ), is flexible, which leads to the large bandgap and difficulty in carrier doping because of the ease of structural relaxation on impurity doping. The coordination number of Ge 4+ ion increases to six in the HP phases ( Fig. 1a,d ), and the decrease of the bandgap is clearly observed as seen in the inset of Figure 3a . The right-hand panel of Figure 4d shows the band alignment of these materials, which was compiled from the calculated DOSs in the left figure of Figure 4d . The CBMs of these oxides are composed of Ge 4 s and O 2p orbitals, and the valence band maximums (VBMs) are usually composed of O 2p orbitals. The differences in the VBM energies are as small as 1 eV, and therefore, the bandgap differences among these Ge oxides are caused primarily by the difference in the CBM energies. Next, we describe the origin of the small bandgap of HP-SrGeO 3 based on the concept of superdegeneracy that prohibits hybridization of relevant orbitals at the Γ point due to the symmetry and the periodicity in a crystal; that is, the transfer and overlap integrals between an s orbital and two sandwiching p x orbitals are exactly zero, which leaves the s - p x bonds nonbonding states at the Γ point [13] , [14] , [15] . The CBMs of conventional Ge-based oxides are high, because the Ge 4 s and O 2p orbitals form covalent chemical bonds and the CBM levels are raised by their resultant anti-bonding nature. However, in HP-SrGeO 3 with cubic perovskite type, the CBMs belong to superdegenerate systems [14] , [15] where the translational symmetry strictly prohibits hybridization between the Ge 4 s and O 2 p orbitals at the Γ point. This is illustrated in the right-bottom figure of Figure 4a . Consequently, the CBM corresponds to a nonbonding state that is exclusively composed of Ge 4 s orbitals and its energy level remains unchanged. Regarding the CBM dispersion, the energy level at the X point (the right-middle figure) is significantly raised, because a Ge 4 s orbital hybridizes with a lobe of an aligned O 2 p orbital forming an anti-bonding orbital. Therefore, HP-SrGeO 3 has a dispersed CB with a width of 7 eV, which results in a deep CBM energy and the small bandgap of 2.7 eV, despite having the largest Ge–Ge interionic distance (0.380 nm) among the four Ge-oxide crystals. The low energy and large dispersion of the CBM in the HP-SrGeO 3 phase makes it possible to realize high-density electron doping and a small effective electron mass in this material. Finally, we describe the large discrepancy between the calculated absorption edge (3.3 eV) and bandgap (2.7 eV) for HP-SrGeO 3 . This discrepancy originates from the fact that HP-SrGeO 3 is an indirect transition-type semiconductor, which is indicated by the band structure shown in Figure 4a . The results obtained in Figures 2d,e and 3 show that the sample has a high density of doped electrons and a high electrical conductivity in addition to transparency (that is, the white colour of the sample seen in the inset of Fig. 2e ). In HP-SrGeO 3 , the high conductivity is caused by the deep CBM, which originates from the small indirect bandgap, and the visible transparency is caused by the large direct bandgap (>3 eV). In summary, we have found that a Ge oxide, cubic SrGeO 3 , is converted to a good electronic conductor by keeping visible transparency. A low CBM energy and a large CB dispersion originating from superdegeneracy in the high symmetry of the cubic perovskite structure make it possible for SrGeO 3 to have both the high conductivity and the high transparency. On the basis of the present finding, we propose that wide-gap oxides with high-symmetry crystal structures and high covalency are potential candidates for new TCOs irrespective of the absence of a large overlap between the vacant s -orbitals of neighbouring metal cations. We expect this to serve as a new design concept for frontier cultivation of TCOs, and it is comparable to a design concept of 'cage conduction band' [10] , [16] , which is derived from the discovery of transparent conductive 12CaO·7Al 2 O 3 (ref. 17 ). Synthesis Polycrystalline samples of SrGeO 3 were prepared using a solid-state reaction from SrCO 3 , GeO 2 and La 2 O 3 . Stoichiometric amounts (SrGeO 3 for undoped, and (Sr 0.95 La 0.05 )GeO 3 for La-doped SrGeO 3 ) of the reagents were mixed and calcined at 1,200 °C for 10 h in air under AP to synthesize the AP-phase SrGeO 3 . The AP-phase samples were subjected to high-pressure reactions at 5.5 GPa and 1,100 °C for 1 h, using a belt-type HP apparatus. AP- and HP-phase GeO 2 (AP-GeO 2 and HP-GeO 2 , respectively) were also synthesized for comparison. Characterization Powder X-ray diffraction patterns were obtained using Cu K α radiation to determine the crystal structure. The cation stoichiometry was confirmed by X-ray energy dispersive spectroscopy with a Hitachi S-4500 SEM equipped with a Kevex Sigma analyser. DC electrical conductivity measurements were carried out by the conventional four-probe method. Seebeck coefficient measurements were performed using the static method. Diffuse reflectance spectra were measured on powder samples over the spectral range of 240–2,600 nm using MgO powder as a reference. The data were transformed to absorbance spectra using the Kubelka–Munk relation. Absolute reflectance spectra were measured in the range from 250–2,500 nm with the spectrophotometer (Hitachi, U-4000) equipped with an absolute specular reflection attachment at an incident angle of 5° from the normal. IR reflectance spectra were measured using mirror-polished samples and a Fourier transform IR spectrometer (Perkin Elmer, Spectrum One). The incident angle was fixed at 20° from the normal and an Al mirror was used as a 100% reflectance standard. Optical dielectric functions were measured by spectroscopic ellipsometry (Jobin-Yvon, UVISEL) at incident/reflection angles of 70° in the photon energy range 0.6–5.0 eV. These data were analysed based on the Drude and Tauc-Lorentz model. Band structure calculation The band structures were calculated by hybrid functional level density functional theory using a code VASP 5.2 (ref. 18 ). We employed PBE0 hybrid functional with a standard mixing parameter of 25% for the exact-exchange term, because we confirmed that it gave a reasonable bandgap for ZnO (3.17 eV for the calculated value and 3.37 eV for the experimental value). Additionally, it gave the closest optical properties to the observed optical properties of the SrGeO 3 samples among the different functionals used, that is, PBE96, PBE0 and HSE [19] , [20] , [21] , [22] . How to cite this article: Mizoguchi, H. et al . A germanate transparent conductive oxide. Nat. Commun. 2:470 doi: 10.1038/ncomms1484 (2011).